Biomimetic block copolymer particles with gated nanopores and ultrahigh protein sorption capacity The design of micro- or nanoparticles that can encapsulate sensitive molecules such as drugs, hormones, proteins or peptides is of increasing importance for applications in biotechnology and medicine. Examples are micelles, liposomes and vesicles. The tiny and, in most cases, hollow spheres are used as vehicles for transport and controlled administration of pharmaceutical drugs or nutrients. Here we report a simple strategy to fabricate microspheres by block copolymer self-assembly. The microsphere particles have monodispersed nanopores that can act as pH-responsive gates. They contain a highly porous internal structure, which is analogous to the Schwarz P structure. The internal porosity of the particles contributes to their high sorption capacity and sustained release behaviour. We successfully separated similarly sized proteins using these particles. The ease of particle fabrication by macrophase separation and self-assembly, and the robustness of the particles makes them ideal for sorption, separation, transport and sustained delivery of pharmaceutical substances. Nature uses molecular self-assembly to construct complex functional structures. Each living cell is surrounded by a self-assembled membrane of phospholipids. These membranes prevent molecules generated inside the cell from leaking out and unwanted molecules from diffusing in [1] . Another typical example of a natural self-assembling system is the viral capsid, which consists of protein subunits that self-assemble into a robust protein coating that protects the viral genome molecules and releases them at the correct moment by a gating mechanism [2] . Although viral vectors have been extensively investigated as promising drug delivery vehicles, their clinical applications have been limited owing to potential risks such as immune recognition and mutagenesis [3] . In the past decade, hierarchical self-assembly inspired by nature has evolved into an effective and practical strategy to fabricate supramolecular structures with transfer or delivery functions in medical applications. Lipid vesicles (liposomes) are relatively easy to make from cheap ingredients. However, they are not very robust since their walls are as thin as the walls of soap bubbles. Synthetic polymer vesicle (polymersome) membranes can also be used as bilayers with improved physicochemical and mechanical properties [4] , [5] , [6] although the level of complexity of such block copolymer (BCP) self-assembled systems is much lower than the level of complexity designed by nature, for example, cell or virus systems ( Supplementary Fig. 1 ). With a few exceptions, the self-assembly of synthetic molecules including BCPs [7] , [8] , surfactants [9] and synthetic peptides [10] , [11] has yielded closed vesicles with limited functionality, whereas greater complexity is needed to develop truly functional biomimetic materials. Here we report for the first time a simple strategy to fabricate micrometre-sized spheres with gated nanopores by BCP self-assembly. Capsules with gated pores have been described before [12] ; in contrast to these capsules our particles are not hollow. They have complex but highly ordered structures with regular and highly dense nanometre-sized pores. Their formation by BCP self-assembly takes hours and involves different stages. We trapped intermediate structures at different times to understand their possible formation mechanism. We found that the particles could be separated easily from various aqueous media via centrifugation. A remarkable property of the particles is their stimulus (pH, ion) responsiveness. Indeed, our tunable nanopores can be used as sensitive gates controlled by pH without any modification. We then tested the particles as potential drug-delivery vehicles. The particles exhibit high loading capacity and sustained release behaviour that might be related to their outer and inner porous structures. Moreover, we used our particles to separate similarly sized proteins (bovine haemoglobin (BHb) 65 kDa, bovine serum albumin (BSA) 66 kDa) in an efficient way by controlling the environmental pH. We envision that when carefully designed, these particles will mimic both the structure and function of sophisticated biological systems ( Supplementary Fig. 2 ), and will thus possess attributes useful for applications in biotechnology, medicine, photoelectric materials and catalysis [13] , [14] . Preparation and characterization of nanoporous particles We used the diblock copolymer polystyrene- b -poly(acrylic acid), PS- b -PAA, as the starting material. Toluene and methanol were chosen as selective solvents for PS and PAA, respectively. Many factors, for example, the composition and concentration of the copolymer, the nature and the content of solvents, and the corresponding block–block and block–solvent χ-parameters (the Flory–Huggins parameter [15] , [16] ), significantly affect the morphology of the material. χ can be roughly estimated by analysing the difference between the solubility parameters ( δ ) of each component. When the values of the solubility parameters for the polymer and the solvent are similar, dissolution of polymer is optimal. As these values diverge, the polymer coils in diluted solutions contract [17] , [18] . In BCPs, the differences in the solubility of each block and solvent will determine which block is preferentially exposed to the solvent. 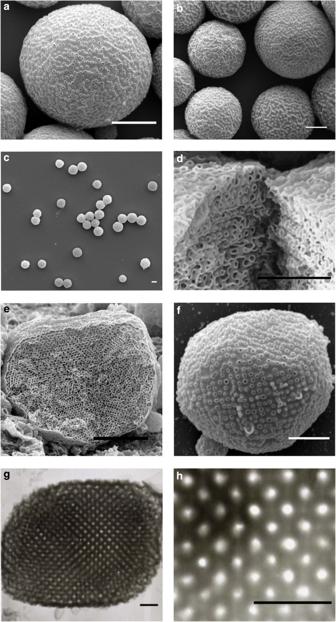Figure 1: SEM and TEM images of spherical particles with regular nanometre-sized pores of high density. (a–c) SEM images of spherical particles at different magnifications. (d,e) Cross-sectional SEM images of the fractured porous particle at different magnifications. (f) Monodispersed nanopores on flat particle surface. (g,h) TEM images of monodispersed nanopores. Scale bars represent 1 μm (a–f) and 200 nm (g,h). Supplementary Table 1 lists the dispersive ( δ d ), polar ( δ p ) and H-bond ( δ H ) contributions of the single solvents, solvent mixtures and copolymer blocks investigated here. ( δ solvent − δ block ) 2 gives a good indication of how strong the interaction between the blocks and the solvent is, with larger values indicating poorer interactions, similarly to recently reported pore formation in PS- b -P4VP BCP membranes [19] . The solubility parameter of a solvent mixture as well as the aggregate morphology can be tuned by changing the solvent composition. To form the porous nanoparticles shown in Fig. 1 , ca . 10 mg of PS- b -PAA was added to a mixture of toluene (0.3 ml) and methanol (0.9 ml). The δ- values of this solvent mixture (1) are also estimated ( Supplementary Table 1 ). Methanol and acrylic acid are much more polar and H-bond forming than is styrene. Differences in the solubility parameters are much larger between styrene blocks and the solvent mixture (( δ p solvent mix1 − δ p S ) 2 =67, ( δ h solvent mix1 − δ h S ) 2 =156) than they are between acrylic acid and the solvent mixture (( δ p solvent mix1 − δ p AA ) 2 =7.8, ( δ h solvent mix1 − δ h AA ) 2 =2.9). The styrene blocks tend not to have contact with the solvents. Figure 1: SEM and TEM images of spherical particles with regular nanometre-sized pores of high density. ( a – c ) SEM images of spherical particles at different magnifications. ( d , e ) Cross-sectional SEM images of the fractured porous particle at different magnifications. ( f ) Monodispersed nanopores on flat particle surface. ( g , h ) TEM images of monodispersed nanopores. Scale bars represent 1 μm ( a – f ) and 200 nm ( g , h ). Full size image Figure 1a–c shows scanning electron microscopy (SEM) images of spherical particles at three different magnifications. We found that the diameter of the obtained particles was around 2 μm and the particles had regular and ordered channels with highly dense and uniform pores perpendicular to the surface. The diameter of the regular pores at the particle surface was ∼ 27 nm as measured in the SEM images under high magnification. The pore density on the surface, as shown in Fig. 1a , was estimated to be around 2.1 × 10 13 pores per square metre. Multilayers with well-ordered nanopores were exposed as the internal structure as shown in the cross-sectional SEM image ( Fig. 1d,e ). A fracture of the internal layers showed that there were larger pores (the average diameter was around 50 nm) inside the particles than on the surface. Interestingly, a highly ordered pattern of monodispersed nanopores was observed on the flat surfaces of some particles ( Fig. 1f ), suggesting that flat surfaces might lose their planarity to reduce energetic stretching at the ridges and evolve into curved surfaces, forming spherical particles. The highly ordered multilayer structures with perpendicular channels were further confirmed by transmission electron microscopy (TEM; Fig. 1g,h ). A phase diagram and a possible formation mechanism A systematic experimental phase diagram of PS 144 - b -PAA 22 in toluene–methanol mixtures as a function of the copolymer concentration and solvent composition is shown in Fig. 2a . All presented structures were observed after stirring for 8 h. Five regions of interest (dense spheres, vesicles, lamellae, tubes and porous particles) were observed. Representative images of morphologies in each region are shown as inset. The predominance of each morphology is governed by the copolymer concentration and methanol/toluene v/v ratio. The phases have been detected in copolymer concentrations below 5 wt%. The diagram pinpoints a relatively narrow regime of porous particles. 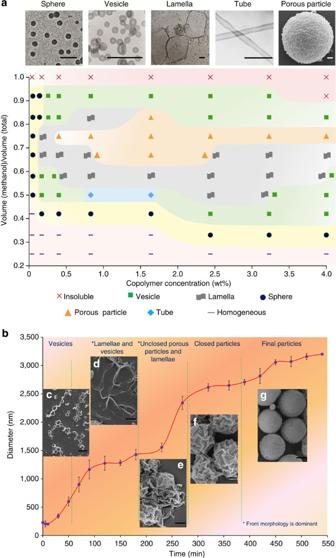Figure 2: Particle formation as function of time, copolymer concentration and solvent composition. (a) Morphological phase diagram of PS144-b-PAA22in toluene–methanol mixtures as a function of copolymer concentration and solvent composition. Five regions of interest were observed—spheres, vesicles, lamellae, tubes and nanoporous particles—as shown in the inset images. Scale bars represent 200 nm. (b) Formation of the nanoporous particles and the changes of hydrodynamic diameter measured by DLS. (c–g), SEM images showing the morphology evolution with time. The scale bars correspond to 1 μm. Figure 2: Particle formation as function of time, copolymer concentration and solvent composition. ( a ) Morphological phase diagram of PS 144 - b -PAA 22 in toluene–methanol mixtures as a function of copolymer concentration and solvent composition. Five regions of interest were observed—spheres, vesicles, lamellae, tubes and nanoporous particles—as shown in the inset images. Scale bars represent 200 nm. ( b ) Formation of the nanoporous particles and the changes of hydrodynamic diameter measured by DLS. ( c – g ), SEM images showing the morphology evolution with time. The scale bars correspond to 1 μm. Full size image Polymer phase diagrams in a binary solvent mixture are characterized by thermodynamic conditions of complete homogeneity (solution), instability and metastability. When the system is brought from homogeneous condition into the instable region, phase separation usually takes place by spinodal decomposition with concentration fluctuations smoothly increasing [20] . Nucleation and growth is the predominant mechanism in the metastable region. When the macromolecular component is an amphiphilic BCP a more complex diagram is obtained reflecting the structures observed in Fig. 2a . Dense spheres are characteristics of nuclei formed by nucleation and growth in the border between metastable and homogeneous region. Nuclei formation requires crossing a free energy barrier. Infinitesimal fluctuation of parameters like density can lead to molecular arrangements corresponding to the thermodynamic concentrations accordingly to those required for keeping the nuclei in equilibrium with the solution with equal probability to grow or dissolve [21] . The free energy stabilizing the nuclei has to overcome the surface energy involved in the formation of the new interface. Density fluctuations alone, depending on the compositions, may not be enough to account for nuclei formation with long-lifetime stability. As proposed by Vekilov [21] , only fluctuations leading to a structure with low enough total final free energy will be stable. Density fluctuation in amphiphilic systems like BCPs can locally favour the formation of mesoscale structures, which could otherwise be found only in homogeneously high concentrated solutions. For PS 144 - b -PAA 22 , as demonstrated in Fig. 2a,b , a rich variety of ordered structures thermodynamically stabilizes the system coexisting with the less diluted solution. The most stable structure is governed by the bend energy, entropic packing restrictions and interaction between blocks and solvent mixtures [22] , [23] . The formation of crew-cut micelle-like aggregates of diblock copolymers in aqueous solutions and their morphology change to cylinders, vesicles and lamellae has been explored and revised by Eisenberg’s group [24] . But the most interesting structures observed in our work are triply periodic continuous minimal surfaces, which can be seen when the porous particle obtained in methanol/toluene solutions are fractured. The morphology is analogous to those theoretically proposed by Schwarz [25] and Schoen [26] with total mean curvature close to zero [27] . The structures are known as Schwarz P and Schoen Gyroid, as shown in Fig. 3d,e . Triply periodic structures have been reported for BCPs in bulk [28] , [29] but not in copolymer solutions analogous to what we report here. Formation of a periodic morphology is believed to alleviate the entropic penalty associated with copolymer segment stretching when assembling in ordered microdomains [28] . Hashimoto et al. [29] proposed the preparation of intercontinuous porous structures by obtaining gyroid morphology in BCP bulk followed by selective degradation of one of the block phases. We are able to obtain a regular periodic porous structure in one step without any selective etching or degradation. 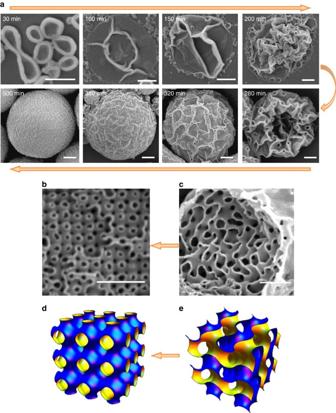Figure 3: SEM images of microparticles. (a) SEM images of a single nanoporous particle formation. Scale bars represent 500 nm. (b–e) Cross-sectional SEM images of the final porous particle with Schwarz P surface (b) formed after 8 h and the intermediate particle with Schoen gyroid structure (c) formed after 5 h. Graphic representations of the Schwarz P surface (d) and the gyroid structure (e). Scale bars represent 500 nm. Figure 3: SEM images of microparticles. ( a ) SEM images of a single nanoporous particle formation. Scale bars represent 500 nm. ( b – e ) Cross-sectional SEM images of the final porous particle with Schwarz P surface ( b ) formed after 8 h and the intermediate particle with Schoen gyroid structure ( c ) formed after 5 h. Graphic representations of the Schwarz P surface ( d ) and the gyroid structure ( e ). Scale bars represent 500 nm. Full size image We followed the kinetics of porous particle formation by dissolving the copolymer in the target solvent composition and extracting samples after different times. The samples were quenched with pure methanol to kinetically trap the intermediate structures. The evolving process of particle formation is shown in Fig. 2b as well as the change of hydrodynamic particle diameters measured by dynamic light scattering (DLS). Additional images for a single porous particle evolution are presented in Fig. 3a . The process follows mainly three steps: (1) vesicles and lamella: density fluctuations lead to local concentrations favouring vesicle formation ( Fig. 2c ). Collapsed vesicle structures similar to ‘Kippah vesicles’, described by Eisenberg [30] and van Hest [31] , are seen in this stage. The vesicles fuse to form lamellas, which are energetically favourable because the total interfacial energy between the aggregates and the solvent outside is reduced. Figure 2d shows lamellas coexisting with vesicles. (2) Lamella to Schoen gyroid [26] transition ( Fig. 2d–f ): at this stage, particles with triply continuous gyroid structures ( Fig. 2f ) were detected. A cross section of the intermediate particle is shown in Fig. 3c , confirming the gyroid morphology. Freestanding lamella can easily lose their morphological stability and exhibit complex configurational changes in response to force, compression, or differential or constrained swelling/shrinkage. No morphological transition happened to the lamellas when stirring was stopped. The transition from lamella to gyroid phases was observed for the first time in self-assembled BCP nanoporous particles. This transition has been mostly previously observed for diblock copolymers in melts [32] , [33] , [34] . (3) Gyroid to Schwarz P structure transition ( Fig. 2f–g ): gyroid and Schwarz P structures are both examples of triply periodic minimal surfaces, which are minimal surfaces that are periodic in all three coordinate directions [35] . Because Schwarz P surface has less surface area than gyroid [28] , the transition from the particles with gyroid surfaces to that with Schwarz P surfaces in the present work is energetically more favourable. The cross section of the porous particle is shown in Figs 1e and 3b . pH-Responsive properties We found that the particles could be easily transferred from various aqueous media via centrifugation. 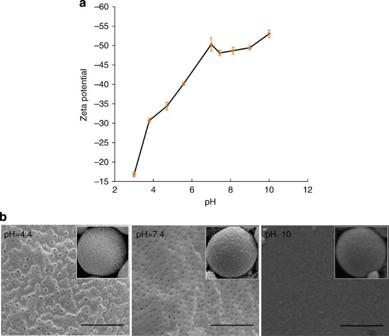Figure 4: ξ Potential and pore size as function of pH. (a) ξ potential of particles versus pH. (b) SEM images of the particles at different pH. With increase of pH, the size of the pores gradually decreases. Scale bars represent 1 μm. Figure 4a indicates how the ξ potential changes as the pH of the buffer solution changes. The ξ potential was below zero at all pH values tested and decreased as the pH increased. Compared with the pore sizes of particles at low pH, the pore size of particles at high pH obviously decreased ( Fig. 4b ). The effect of pH on the morphology is mainly due to the change in the swelling and electrostatic repulsion generated by ionization of the PAA blocks. The carboxylic acid units were deprotonated at high pH and the PAA segments stretched to minimize the charge repulsion, transforming the pore into a pH-sensitive gate without affecting the overall spherical shape of the particle. The effect is opposite to that observed in recently reported stimuli-responsive PS- b -P4VP isoporous membranes [36] , [37] . Figure 4: ξ Potential and pore size as function of pH. ( a ) ξ potential of particles versus pH. ( b ) SEM images of the particles at different pH. With increase of pH, the size of the pores gradually decreases. Scale bars represent 1 μm. Full size image It is worth noting that these particles could be lyophilized without adding any cryoprotective agent and the resulting dried powder was easy to redisperse. The morphology of the particles after lyophilization and redispersion ( Supplementary Fig. 3 ) did not change much and remained similar to that of the original particles. This is very favourable for applications in drug delivery and nanoreactors. Similarly sized protein separation Size-based separation of proteins can be carried out by ultrafiltration membrane systems when the proteins are significantly different in size [38] , [39] . However, separation of similarly sized proteins with the commercially available membranes is not possible [40] . Here we tested whether our porous particles could separate similarly sized proteins with high selectivity. To determine whether our porous particles could separate proteins, we chose two proteins with different isoelectric points (pI): BSA (pI=4.7, molecular weight (MW)=67 kDa, diameter=6.8 nm) and immunoglobulin-γ (IgG, pI=7.3, MW=150 kDa, diameter=14 nm), fluorescently labelled with Alexa 488 and Alexa 546 (Molecular Probes), respectively. BSA and IgG are too close in size (there is a twofold difference in their MW) to be separated efficiently via conventional dialysis membrane processes [41] (dialysis membrane manufacturers recommend that there be at least a 10-fold MW difference between separable proteins). A critical parameter that can influence separation through nanopores is the charge of the protein. When the pH value of a buffer solution is exactly equal to the pI of a protein, the surface charge of the protein is neutral. At a pH above the pI, the protein is negatively charged; at a pH below the pI, the protein is positively charged. Proteins are large biomolecules and can thus be heavily charged (BSA’s net charge is −13 at pH 7) [42] . Strong electrostatic interactions between proteins and charged particles were therefore expected. We monitored the separation of fluorescently labelled BSA (denoted as BSA*) and fluorescently labelled IgG (denoted as IgG*) using our porous particles at pH 5.8 simultaneously on two channels of a fluorescence microscope ( Supplementary Fig. 4a ). The IgG molecules carried positive charges, which caused strong electrostatic attraction and adsorption into the negatively charged particles. Highly efficient separation could be clearly observed in laser scanning confocal microscopy (LSCM) images within 2 min. 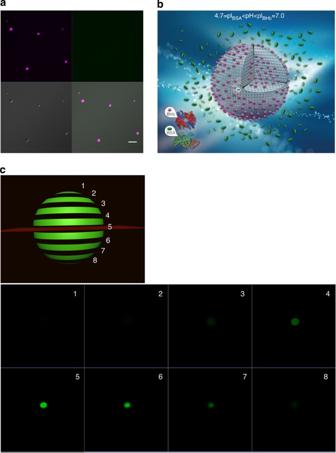Figure 5: Selective separation of similarly sized proteins using the nanoporous particles. (a) LSCM images (taken from the same field of microscope) of spherical particles mixed with two fluorescently labelled proteins (BHb* and BSA*, appear magenta and green in the fluorescence images, respectively). Top left, fluorescence image from channel 1 (magenta) shows BHb*-encapsulated particles; top right, fluorescence image from channel 2 (green) shows that no BSA* was adsorbed into the particles; bottom left, transmission image; bottom right, overlay of the three images, showing that only BHb* was adsorbed into the negatively charged particles. This selective separation of BSA* and BHb* at pH 5.8 was confirmed by simultaneous two-colour imaging of particles. Scale bars represent 10 μm. (b) Schematic of the selective separation process of BSA (green ellipsoid) and BHb (magenta sphere) using the particle at pH 5.8. (c) A single particle was imaged byz-slice imaging. The cross-sectional pictures are shown in series from the top of the particle (top left fluorescence image 1) to the bottom (bottom right fluorescence image 8), clearly indicating the three-dimensional, non-hollow nature of the structure. The imaged particle is about 2 μm in diameter. Figure 5a,b shows a similar experiment using fluorescently labelled BSA and BHb at pH 5.8. BSA and BHb have nearly identical molecular weights (BHb 65 kDa; BSA 66 kDa), making them more difficult to separate. However, BSA has a lower isoelectric point (pI=4.7) than BHb (pI=7.0). Similar to the experiment with BSA and IgG, positively charged BHb was rapidly adsorbed into our porous particles while negatively charged BSA was electrostatically repelled. The negative charge of the particles increased the selectivity of BHb over BSA. Because the electrostatic interactions between the proteins and the particles occurred throughout the particles, not only at their surfaces, the particles offered sufficient electrostatic interaction space for selective separation. Figure 5: Selective separation of similarly sized proteins using the nanoporous particles. ( a ) LSCM images (taken from the same field of microscope) of spherical particles mixed with two fluorescently labelled proteins (BHb* and BSA*, appear magenta and green in the fluorescence images, respectively). Top left, fluorescence image from channel 1 (magenta) shows BHb*-encapsulated particles; top right, fluorescence image from channel 2 (green) shows that no BSA* was adsorbed into the particles; bottom left, transmission image; bottom right, overlay of the three images, showing that only BHb* was adsorbed into the negatively charged particles. This selective separation of BSA* and BHb* at pH 5.8 was confirmed by simultaneous two-colour imaging of particles. Scale bars represent 10 μm. ( b ) Schematic of the selective separation process of BSA (green ellipsoid) and BHb (magenta sphere) using the particle at pH 5.8. ( c ) A single particle was imaged by z -slice imaging. The cross-sectional pictures are shown in series from the top of the particle (top left fluorescence image 1) to the bottom (bottom right fluorescence image 8), clearly indicating the three-dimensional, non-hollow nature of the structure. The imaged particle is about 2 μm in diameter. Full size image It is worth noting that BSA could also be loaded into the particles when the pH value is below the pI of BSA ( Supplementary Fig. 4b ). Figure 5c shows the cross-sectional pictures of a single particle loaded with BSA at pH 4.4. In this case, electrostatic attraction between the BSA molecules and particles occurs as a result of their opposite charges. The images indicate that the circles are solid rather than hollow, suggesting that the positively charged BSA was not only adsorbed onto the surface of the particles but it also was drawn inside the particles through the nanopores. Separation experiments with fluorescently labelled proteins revealed that our porous particles had enough capacity to load even large protein molecules. Given the hours-long passage times of molecules through thick membranes [43] , our particles demonstrate significant advantages in effective bioseparation within minutes, even for similarly sized proteins with opposite charges. This is very favourable for applications in high-speed protein chromatography. Drug loading tests of the particles Bioactive agents such as proteins or nucleic acids are usually too polar to enter cells directly and hence require carriers for cellular delivery [44] . A high loading capacity is important to reduce the dose of the carrier in clinical practice. Because of the porous structure and the charged nature of our particles, they may be promising candidates to be drug carriers with high loading capacities. We loaded BHb and IgG molecules into the particles and observed a surprisingly high loading capacity for both proteins. For example, the maximum BHb loading capacity at pH 5.8 is as high as 1,600% after 3 days (that is, a 1-mg particle can load about 16.0 mg of BHb). More remarkably, the loading capacity of IgG at this pH was >3,000%, which is at least 50 times larger than the loading capacity of the protein in polysaccharide colloidal particles [45] and about 200 times larger than the loading capacity of the protein in micelles assembled by a BCP [46] . We attribute the main driving force of this loading process to the strong electrostatic interactions between the charged proteins and the particles. In addition, the high porosity of the particles has crucial effects on the high-capacity adsorption process. First, the highly dense nanopores on the surface and inside the particles become channels for the proteins to enter inside the particles where they can make full use of the internal structure. Second, the size of nanopores is close to that of the protein molecules, which made it difficult for the proteins to leach out once they entered. The Brunauer–Emmett–Teller (BET) surface area and total pore volume were estimated to be 149 m 2 g −1 and 0.46 cm 3 g −1 , respectively. The high surface area and volume from BET result is consistent with the high loading capacity of the porous particles. The pore size distribution ( Supplementary Fig. 5 ) was calculated from N 2 adsorption isotherm using density functional theory method, and matches well with the SEM images. The pore volume percent is estimated to be about 49.5% in present work. Sustained drug release behaviour Besides loading of a drug, release of the drug is another important parameter in determining the efficacy [47] of a drug within a therapeutic range [48] , [49] . The binding of the proteins in our porous particles is through electrostatic interaction; the release process would have to be a combination of desorption and diffusion, and would be dependent on the pH of the environment. We observed a controlled and constant release of entrapped IgG antibodies by our particles at different pH without physical and chemical stresses over a period of 30 days ( Fig. 6a ). The release processes taking place in the case of IgG are complex because both the protein charge and the pore size of the particle are sensitive to changes in pH. For instance, IgG is negatively charged at pH 9 and would thus be repelled from negatively charged particles. The release rate of the protein was constant over time irrespective of the concentration of the protein. We interpret this to be a consequence of single-file diffusion [50] , [51] , which is known as the best long-term controlled delivery system for protein drugs. When pore sizes are controlled so that two or more diffusing molecules are not allowed to pass through the pores simultaneously, protein-based drugs are released by single-file diffusion through the pores. On the other hand, an increase in pH would strengthen the repulsion between charged IgG and the particles, thus increasing the release rate ( Fig. 6a ). 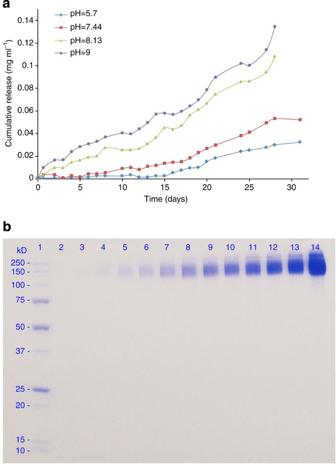Figure 6: Protein drug loading and sustained release. (a) Concentration of the released protein versus time at different pH. (b) The results of SDS–PAGE analysis ofin vitroreleased IgG up to 30 days and IgG stock solution. Lane 1:5 μl protein molecular weight standards; lane 2: blank; lane 3–13: 10 μl released protein samples collected after 0.5, 3, 6, 8, 10, 12, 15, 18, 22, 26 and 30 days, respectively; lane 14: 2.5 μl initial stock solution of IgG. Figure 6: Protein drug loading and sustained release. ( a ) Concentration of the released protein versus time at different pH. ( b ) The results of SDS–PAGE analysis of in vitro released IgG up to 30 days and IgG stock solution. Lane 1:5 μl protein molecular weight standards; lane 2: blank; lane 3–13: 10 μl released protein samples collected after 0.5, 3, 6, 8, 10, 12, 15, 18, 22, 26 and 30 days, respectively; lane 14: 2.5 μl initial stock solution of IgG. Full size image We used one-dimensional SDS–polyacrylamide gel electrophoresis (PAGE) gel electrophoresis analysis to confirm that the released protein was intact without denaturation after days or even months. Released IgG was detected at the same position with its molecular weight intact as shown in Fig. 6b , indicating that IgG retained its original active structure after loading and release. BCP microspheres with stimuli-responsive nanopores and very high specific protein adsorption could be manufactured by macrophase separation and self-assembly. The final spherical particles were obtained after stirring PS- b -PAA in a methanol/toluene mixture for 8 h. By adding a large excess of methanol at different time intervals intermediate structures could be kinetically trapped and isolated. This helped to understand the formation mechanism of the unique superstructure of the porous microspheres. The transitions from lamella to gyroid and then to Schwarz P structure were reported here for the first time in self-assembled BCP particles in solutions. Owing to the internal porous structure with numerous binding sites, the protein loading capacity of the particles is at least two orders of magnitudes higher when compared with BCP micelles. One milligram of particles could adsorb 30 mg of IgG. Depending on the external pH the entrapped protein could be released with a constant rate over a period of 30 days. These particles have also been used for selective separations of similarly sized proteins in the present work. When carefully designed these particles will mimic both the structure and function of more sophisticated biological systems and will thus possess attributes useful for applications in biotechnology, pharmacy and medicine. Microparticle preparation PS- b -PAA BCP P4002-SAA (PS 144 - b -PAA 22 , M n =16,600 g mol −1 , PDI=1.10) was purchased from Polymer Source, Inc., Canada. Toluene and methanol were supplied by Fisher Scientific. To prepare the nanoporous particles, we added 10 mg PS- b -PAA to a mixture of 0.3 ml toluene and 0.9 ml methanol. The mixture was magnetically stirred (1,000 r.p.m.) at room temperature for 8 h (or for varying times for the kinetic studies). Then, a fivefold larger amount of methanol was added to dilute the resulting solution. The resulting suspension was centrifuged at 14,000 r.p.m. for 15 min. Finally, the sediments of the obtained particles were freeze-dried and redispersed into buffer solutions with different pH. All the buffer solutions were adjusted to desired pH values by mixing different amounts of potassium dihydrogen phosphate (KH2PO4) and disodium hydrogen phosphate (Na2HPO4) (both from Fluka) in Milli-Q water and using these solutions within 3 days of preparation. Phosphate buffer saline solutions maintaining different external pH with low ionic strength (I=0.01 M) were used in the experiments [38] . Dynamic light scattering DLS measurements were performed with a Malvern NanoZS Zetasizer equipped with a 633 nm He–Ne laser. The ξ potential of the samples was obtained with Zetaplus. All DLS measurements were done with a laser wavelength of 658.0 nm and an incident angle of 90° at 25 °C. For each sample, 15 runs of 10 s were performed, with three repetitions for all the BCP particles. Electron microscopy Scanning electron microscopy: To prepare the samples for SEM, a drop of the dilute solution was dropped onto the silicon wafers. Before coating, the silicon substrates were cleaned in a bath of 100 ml of 80% H 2 SO 4 , 35 ml of H 2 O 2 and then 20 ml of Milli-Q water for 15 min at 80 °C. The silicon surface was then dried with compressed nitrogen gas. The coated substrates were then dried in air and stayed at room temperature for 1 day. To avoid charging problems, the samples were sputter coated with gold for 60 s at 20 mA current in an argon atmosphere. The samples were then transferred to an SEM stage and observed on FEI Quanta 600 and Helios 400 S microscopes at 30 kV. Transmission electron microscopy: TEM was performed on a JEOL JEM-1011 microscope operating at an acceleration voltage of 100 kV. The dilute samples were deposited on a carbon-coated copper grid. After 10 min, excess solution was removed using a strip of filter paper. The samples were allowed to dry in air at room temperature before observation. Cryo-field emission SEM (Cryo-FESEM): low-temperature experiments were carried out using a Quorum PP2000T cryo-transfer system (Qurorum Technologies, Newhaven, UK) that was fitted to an FEI Nova Nano630 SEM with a field-emission electron source and through-lens electron detectors. A small amount of BCP solution was dropped on the specimen holder. The sample holder, attached to a transfer rod, was then rapidly plunged into liquid-nitrogen slush, transferred under vacuum to the preparation chamber precooled to −180 °C, and allowed to equilibrate for 10 min. Then sample temperature was raised to −160 °C. To avoid charging problem, the sample temperature was then reduced to −135 °C and the sample was sputter coated with gold–palladium for 90 s at a 5 mA current in an argon atmosphere. The sample was then transferred to an SEM cryo stage, which was held at −140 °C. Fluorescence labelling and protein separation Globulin-γ (IgG, 150 kDa), BSA (66 kDa) and BHb (65 kDa) are from Sigma Co. They were used as received with no further purification. For the protein separation experiments, BSA, BHb and IgG were labelled with Alexa Fluor 488, 647 and 546 dyes (Molecular Probes), respectively. The dyes react with primary amines, forming stable covalent bonds. Each labelled protein was separated from unincorporated dye with the purification resin packed in the column provided in the labelling kit. Protein concentration and degree of labelling was calculated by measuring absorbances with a NanoDrop 2000/2000c Spectrophotometer (Thermo Fisher Scientific) using extinction coefficients provided by the dye manufacturer. This analysis showed that these proteins were all labelled with five moles of dye per mole of protein. In the microscope, this yielded similar fluorescence intensity for each species at the same concentration. In the mixed protein separation experiments, the initial concentrations of proteins were 2.0 mg ml −1 each. Protein mixture (10 μl) and 10 μl particle solution (1 mg ml −1 ) were mixed and sandwiched between a glass slide and a cover-glass, and imaged by LSCM. The microscope (Zeiss LSM 710) was equipped with a × 60 or × 100 oil immersion objective. ZEN 2009 software (Carl Zeiss Microscopy, GmbH) was used to collect and orient the imaging data including the z-slices of a single particle loaded with fluorescently labelled proteins. Measurement of protein loading capacity and protein release Pure particle (1 mg) was mixed with a protein solution at a known concentration. The mixed solution was stirred gently to allow protein absorption into the particles to reach isothermal equilibrium. The drug loading capacity of particles was determined by separating the particles from the buffer solution containing free protein through centrifugation (10,000 r.p.m., 10 min). The amount of free protein in the supernatant was determined by a NanoDrop 2000/2000c Spectrophotometer. The release of the proteins from purified protein-loaded particles with a known concentration was performed in buffer solutions of different pH. The released protein was sampled at defined time periods and their concentrations were measured using a NanoDrop 2000/2000c Spectrophotometer. PAGE analysis and gel staining Laemmli (SDS–PAGE) sample loading buffer, 10 × Tris/glycine/SDS electrophoresis migration buffer, 4–20% Mini-PROTEAN TGX Precast Gel, Precision Plus Protein Unstained Standards (10–250 kDa) and Bio-Safe colloidal Coomassie brilliant blue G-250 protein staining solution were purchased from Bio-Rad (USA). One part of the sample was diluted with one part of the Laemmli sample buffer. The SDS–PAGE was then carried out on a 4–20% precast polyacrylamide gel in a Mini-PROTEAN Tetra Cell (Bio-Rad). The migration of the proteins occurred at constant voltage of 100 V with initial current of 20 mA gel −1 and at 1 W for about 1.5 h in migration buffer. After electrophoresis, the gel was stained with colloidal Coomassie blue G250 for 2 h with gentle agitation and then washed in Milli-Q water until the background was clear. How to cite this article: Yu, H. et al. Biomimetic block copolymer particles with gated nanopores and ultrahigh protein sorption capacity. Nat. Commun. 5:4110 doi: 10.1038/ncomms5110 (2014).